Retinoid X receptor α attenuates host antiviral response by suppressing type I interferon The retinoid X receptor α (RXRα), a key nuclear receptor in metabolic processes, is downregulated during host antiviral response. However, the roles of RXRα in host antiviral response are unknown. Here we show that RXRα overexpression or ligand activation increases host susceptibility to viral infections in vitro and in vivo, while Rxra −/− or antagonist treatment reduces infection by the same viruses. Consistent with these functional studies, ligand activation of RXR inhibits the expression of antiviral genes including type I interferon (IFN) and Rxra −/− macrophages produce more IFNβ than WT macrophages in response to polyI:C stimulation. Further results indicate that ligand activation of RXR suppresses the nuclear translocation of β-catenin, a co-activator of IFNβ enhanceosome. Thus, our studies have uncovered a novel RXR-dependent innate immune regulatory pathway, suggesting that the downregulation of RXR expression or RXR antagonist treatment benefits host antiviral response, whereas RXR agonist treatment may increase the risk of viral infections. Retinoid X receptors (RXRs) have been implicated in the control of a variety of physiological processes including cell differentiation, lipid and glucose metabolism and immune responses [1] , [2] , [3] , [4] . They occupy a central position in the nuclear hormone receptor (NR) superfamily, because they not only act as homodimers but are also essential heterodimeric partners of many other NR family members, such as retinoic acid receptor (RAR), vitamin D receptor (VDR), thyroid receptor, liver X receptor (LXR), peroxisome proliferator-activated receptor (PPAR), pregnane X receptor and farnesoid X receptor [5] , [6] . Heterodimerization with partners raises the possibility of pleiotropic RXR signalling, different RXR isotypes and their unique expression increase the complexity of the RXR-controlled transcriptional programs. Mammalian tissue express three RXR isotypes, RXRα, RXRβ and RXRγ, which have specific tissue distributions and expression patterns during development [6] , [7] , [8] , [9] , [10] , [11] . RXRα is the dominant and the most functionally important RXR isotype in myeloid cells, especially macrophages [12] , [13] . All RXR isotypes can be activated by natural and synthetic ligands. The vitamin A derivative, retionid 9-cis-retinoic acid (9cRA), is identified as a high-affinity ligand for RXR [14] , [15] . Endogenous fatty acids such as docosahexaenoic acid, oleic acid and phytanic acid, also activate RXR [7] . Synthetic RXR-specific ligands, called rexinoids, are exemplified by LG100268 (LG268), AGN194204, as well as Targretin (bexarotene), which is a pan-RXR agonist used clinically for the treatment of T-cell lymphoma [15] , [16] , [17] . RXRs regulate the integration of macrophage immune functions and lipid metabolism by controlling apoptotic cell uptake, β-amyloid clearance, inflammation, pathogen killing, cholesterol transport and lipid handling. Alterations in these RXR-mediated processes cause diseases such as atherosclerosis, neurodegeneration, autoimmunity and disorders of the immune response [4] , [11] . We previously showed that RXRα expression was significantly suppressed during host defence against viral infections. Downregulation of RXRα decreases the ability of RXR-dependent hepatic detoxification and thus enhances bile acid- and aspirin-induced hepatotoxicity, which provides evidence that alteration of RXR expression plays a role in the pathogenesis of metabolic disease such as Reye’s syndrome [18] . The crosstalk between RXR and inflammatory responses in macrophages has been extensively studied. Ligand activation of LXR–RXR heterodimer inhibits Toll-like receptor-triggered iNOS, interleukin (IL)-1β, COX2 and IL-6 production [19] . In lipopolysaccharide-stimulated macrophages, ligand activation of RAR–RXR heterodimer reduces synthesis of inflammatory cytokines, IL-12 and tumour necrosis factor-α, and increases the expression of anti-inflammatory cytokine, IL-10 (refs 20 , 21 ). RXRα also controls innate inflammatory responses through the upregulation of the chemokine CCL6 and CCL9 (ref. 13 ). Defect of LXR–RXR signalling increases host susceptibility to Listeria monocytogenes infection [22] . Activation of VDR–RXR leads to the induction of cathelicidin and defensin beta 4 genes, which are essential in combating Mycobaterium tuberculosis [23] . While RXR and inflammatory responses are evidently connected, our previous study implicated a relationship between the host antiviral response and RXRα [18] . It is still unclear whether downregulation of RXRα during viral infection plays a role in the overall host antiviral response. Meanwhile, considering that RXRs regulate the expression of inflammatory cytokines, anti-inflammatory cytokines, and chemokines, it is an interesting issue whether RXRs also modulate the production of type I interferon (IFN) in macrophages. The innate cellular antiviral response involves numerous signalling pathways that generally lead to the induction of type I IFN. Briefly, viral nucleic acids are recognized by pathogen recognition receptors, such as Toll-like receptor, RIG-I, MDA5, IFI16 and cGAS [24] , [25] . These sensors trigger pathways that lead to the activation of tank-binding kinase 1 (TBK1), phosphorylation and nuclear translocation of IFN regulatory factor 3 (IRF3), which subsequently drives type I IFN transcription [24] , [25] , [26] . Type I IFN induces multiple antiviral genes expression through the Jak-Stat1/2 pathway. Some genes, like ISG15, GBP1 and OAS2, directly inhibit viral lifecycle processes [27] . Others like IRF1, IRF7 and the viral nucleic acid sensors (RIG-I and MDA5) further amplify the IFN response [24] , [25] . Recent studies have indicated that β-catenin acts as a co-activator in the IFNβ enhanceosome and synergistically activate IFNβ transcription during host antiviral response [28] , [29] . Sendai virus, vesicular stomatitis virus (VSV), and herpes simplex virus-1 (HSV-1) infections trigger host β-catenin nuclear translocation by activating β-catenin phosphorylation and deacetylation [29] , [30] , [31] . The relationship of these pathways critical in host antiviral response and RXR remains unknown. In this study, we demonstrate that RXRα attenuates host antiviral response by inhibiting type I IFN production and its downstream IFN-stimulated genes (ISGs) expression. We also provide evidence that the suppression of β-catenin nuclear translocation accounts for the downregulation of antiviral genes by RXR signalling. These results illustrate a molecular crosstalk between host antiviral response and metabolic nuclear receptors, suggesting that the downregulation of RXRα expression in response to viral infection is beneficial for optimal type I IFN production and host antiviral immunity. Antiviral immune response suppresses RXRα expression Our previous gene expression profile has shown that VSV infection downregulates RXRα expression in liver [18] . Further studies have indicated that TLR3- or TLR4-activated macrophages suppress RXRα expression in an IRF3-depedent but IFN-independent manner [18] . To verify the previous conclusions, we tried different viral infection models in bone marrow-derived macrophages (BMMs). BMMs were infected with RNA virus, VSV, and DNA viruses, HSV-1 and murine gamma herpes virus (MHV68). Quantitative PCR (qPCR) results indicated that infections with both RNA and DNA viruses led to significant downregulation of RXRα expression ( Fig. 1a ). To exclude certain viral components, such as viral inhibitory noncoding RNAs and proteins, suppressing host RXRα expression, the cells were transfected with polyI:C and polydA:dT,which mimic RNA and DNA viral infections, respectively. We observed that transfection with polyI:C and polydA:dT downregulated RXRα RNA and protein expression in BMMs ( Fig. 1b,c ). These experiments suggest that viral infection suppresses RXRα expression in BMMs and this suppression is due to the host antiviral response. 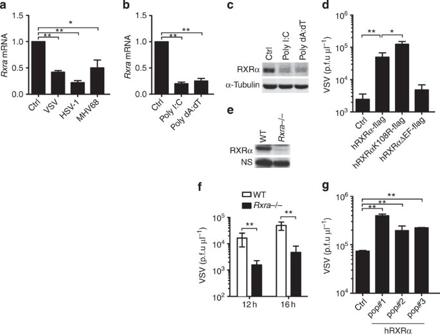Figure 1: Host susceptibility to VSV infection after altering RXRα expression. (a) qPCR detection ofRxramRNA in BMMs infected by VSV for 4 h, HSV-1 or MHV68 for 8 h (MOI=1). (b) qPCR detection ofRxramRNA in BMMs transfected with 1 μg ml−1polyI:C or polydA:dT for 4 h. (c) Immunoblot of RXRα protein in BMMs transfected with 1 μg ml−1polyI:C or polydA:dT for 8 h. (d) RAW264.7 cells stably transfected with pBABE-empty vector (Ctrl), pBABE-hRXRα-flag vector (hRXRα-flag), RXRα sumoylation site mutant (hRXRαK108R-flag) and RXRα LBD-AF2-domain-deficient mutant (hRXRαΔEF-flag). These cells were infected by VSV (MOI=0.01). Supernatants were collected at 14 h.p.i and viral titre was quantified by plaque assay. (e) Immunoblot of RXRα protein in WT andRxra−/− F9 cells. (f) WT orRxra−/− cells were infected by VSV (MOI=0.01) and the viral titre of supernatant was quantified at indicated time point by plaque assay. (g)Rxra−/− F9 cells were reconstituted with pBABE-hRXRα (hRXRα) or pBABE-empty vector (Ctrl) by retroviral infection. Three independent hRXRα-overexpressing populations (pop#1–3) were made, these cells were infected by VSV (MOI=0.01). Supernatants were collected at 12 h.p.i and the viral titre was quantified for by plaque assay. Data ofa,b,d,f,gare shown as mean±s.d. (n=3) of one representative experiment, similar results were obtained in three independent experiments. *P<0.05 and **P<0.01 (Student’st-test). Data ofcandeare representative of three independent experiments. See alsoSupplementary Fig. 7of uncropped blot ofcande. Figure 1: Host susceptibility to VSV infection after altering RXRα expression. ( a ) qPCR detection of Rxra mRNA in BMMs infected by VSV for 4 h, HSV-1 or MHV68 for 8 h (MOI=1). ( b ) qPCR detection of Rxra mRNA in BMMs transfected with 1 μg ml −1 polyI:C or polydA:dT for 4 h. ( c ) Immunoblot of RXRα protein in BMMs transfected with 1 μg ml −1 polyI:C or polydA:dT for 8 h. ( d ) RAW264.7 cells stably transfected with pBABE-empty vector (Ctrl), pBABE-hRXRα-flag vector (hRXRα-flag), RXRα sumoylation site mutant (hRXRαK108R-flag) and RXRα LBD-AF2-domain-deficient mutant (hRXRαΔEF-flag). These cells were infected by VSV (MOI=0.01). Supernatants were collected at 14 h.p.i and viral titre was quantified by plaque assay. ( e ) Immunoblot of RXRα protein in WT and Rxra −/− F9 cells. ( f ) WT or Rxra −/− cells were infected by VSV (MOI=0.01) and the viral titre of supernatant was quantified at indicated time point by plaque assay. ( g ) Rxra −/− F9 cells were reconstituted with pBABE-hRXRα (hRXRα) or pBABE-empty vector (Ctrl) by retroviral infection. Three independent hRXRα-overexpressing populations (pop#1–3) were made, these cells were infected by VSV (MOI=0.01). Supernatants were collected at 12 h.p.i and the viral titre was quantified for by plaque assay. Data of a , b , d , f , g are shown as mean±s.d. ( n =3) of one representative experiment, similar results were obtained in three independent experiments. * P <0.05 and ** P <0.01 (Student’s t -test). Data of c and e are representative of three independent experiments. See also Supplementary Fig. 7 of uncropped blot of c and e . Full size image Alteration of RXRα expression affects VSV infection Alteration of RXRα expression causes numerous metabolic and immune diseases [11] , [18] . To test whether alteration of RXRα expression affects host antiviral response, we performed in vitro infections of hRXRα-overexpressing and Rxra−/− cell lines with VSV and quantified the viral titres in the supernatant of the infected cells by plaque assay. First, we stably overexpressed human RXRα and two RXRα mutants in a macrophage cell line, RAW264.7 cells ( Supplementary Fig. 1a,b ). Overexpression of wild-type (WT) human RXRα made the cells much more susceptible to VSV infection ( Fig. 1d ). The lysine-108 residue within the RXRα AF1 domain mediates RXRα sumoylation during ligand activation, which negatively regulates the transcriptional activity of RXRα and the activity of its heterodimeric complex with RARα and PPARγ [32] . Prevention of RXRα sumoylation by Lys-to-Arg mutation led to modest increase of VSV infection ( Fig. 1d ). However, deletion of the ligand binding/dimerization domain and helix 12 (AF2) of RXRα abolished the ability of RXR to increase host susceptibility to VSV infection, suggesting that the ligand-independent RXRα mutant is not sufficient to affect the host antiviral response ( Fig. 1d ). Next, we took advantage of WT and Rxra−/− F9 embryocarcinoma cells, which have been extensively used to study the function of RXRs in retinoid signalling [33] , [34] ( Fig. 1e ). When these cells were infected with VSV, the viral titre was lower in the supernatant of Rxra−/− F9 cells compared with that of the WT cells ( Fig. 1f ). To confirm that less VSV infection was specifically due to deficiency of RXRα, we rescued the Rxra−/− F9 cells with hRXRα ( Supplementary Fig. 1c ) and found that hRXRα reconstitution led to an increase in the VSV titre after infection compared with control ( Fig. 1g ). Together, the overexpression of RXRα increases host susceptibility to VSV infection and knockout of RXRα decreases host susceptibility to VSV infection. Ligand activation of RXR promotes VSV infection Ligand binding to RXR is required for its downstream signalling and full activation. 9cRA is a high-affinity ligand for RXR and RAR. HX531 is a synthetic RXR antagonist, which could inhibit the activation of both RXR homodimer and RXR–RAR heterodimer [35] . To investigate whether ligand activation of RXR affects host susceptibility to viral infection, RAW264.7 cells were pretreated with 9cRA and HX531 overnight, and subsequently infected with green fluorescent protein (GFP)-expressing VSV (VSV-GFP), which allows the visualization of viral infection by fluorescence microscopy. Apparently, there was more VSV-GFP in the 9cRA-treated cells and less VSV-GFP in the HX531-treated cells than the control dimethylsulphoxide (DMSO)-treated cells ( Supplementary Fig. 2a ). The plaque assay data also indicated that 9cRA treatment promotes VSV infection in a dose-dependent manner and HX531 treatment enhanced host cells against VSV infection ( Fig. 2a and supplementary Fig. 2b ). We tried other two synthetic RXR-specific agonists, LG268 and AGN194204. Significant higher VSV titre was detected in the supernatant of LG268- and AGN194204-treated cells, which indicated that both of them increased host susceptibility to VSV infection as 9cRA ( Fig. 2b ). Combination of AGN194204 treatment and hRXRα overexpression in RAW264.7 further increased VSV infection ( Supplementary Fig. 2c ). In F9 cells, treatment with AGN194204 promoted VSV infection in WT cells, but not in Rxra −/− cells ( Fig. 2c ). However, after we reconstituted hRXRα into Rxra −/− F9 cells, hRXRα-reconstituted cells were infected more VSV than control cells, and AGN194204 treatment further increased host susceptibility to VSV infection ( Fig. 2d ). 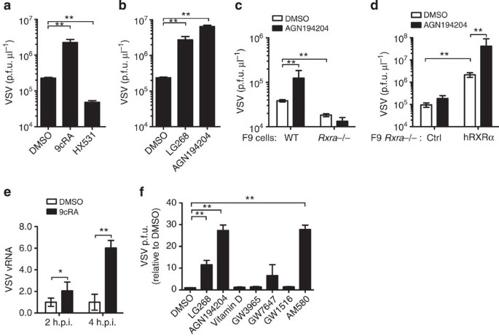Figure 2: Host susceptibility to VSV infection after ligand activation of RXR. (a) RAW264.7 cells were pretreated with DMSO, 9cRA (100 nM) and HX531 (1 μM) for 16 h and infected by VSV-GFP (MOI=0.01). The supernatant was collected at 14 h.p.i and the viral titre was quantified by plaque assay. (b) RAW264.7 cells were pretreated with DMSO or RXR-specific synthetic ligands, LG268 (100 nM) and AGN194204 (100 nM) for 16 h. The cells were subsequently infected by VSV (MOI=0.01) and the supernatant was collected at 14 h.p.i. The viral titre was quantified by plaque assay. (c) WT andRxra−/− F9 cells were pretreated with DMSO or AGN194204 (100 nM) for 16 h and subsequently infected with VSV (MOI=0.01). The viral titre of supernatants was quantified by plaque assay at 12 h.p.i. (d)Rxra−/− F9 cells stably transfected with pBABE-empty vector (Ctrl) or pBABE-hRXRα (hRXRα) were treated with DMSO or AGN194204 (100 nM) and infected with VSV (MOI=0.01). The viral titre of supernatants was quantified by plaque assay at 12 h.p.i. (e) RAW264.7 cells were pretreated with DMSO or 9cRA (100 nM) for 16 h and infected by VSV (MOI=0.01), relative genomic VSV RNA was quantified at 2 and 4 h.p.i. (f) RAW264.7 cells were pretreated with DMSO, RXR agonist LG268 (100 nM), AGN194204 (100 nM), VDR agonist Vitamin D (100 nM), LXR agonist GW3965 (100 nM), PPARα agonist GW7647 (100 nM), PPARδ agonist GW1516 (100 nM) or RAR agonist AM580 (100 nM) for 16 h and subsequently infected by VSV (MOI=0.01). The supernatants were collected at 14 h.p.i and viral titre was detected by plaque assay. Data are shown as mean±s.d. (n=3) of one representative experiment, similar results were obtained in three independent experiments. *P<0.05 and **P<0.01 (Student’st-test). Figure 2: Host susceptibility to VSV infection after ligand activation of RXR. ( a ) RAW264.7 cells were pretreated with DMSO, 9cRA (100 nM) and HX531 (1 μM) for 16 h and infected by VSV-GFP (MOI=0.01). The supernatant was collected at 14 h.p.i and the viral titre was quantified by plaque assay. ( b ) RAW264.7 cells were pretreated with DMSO or RXR-specific synthetic ligands, LG268 (100 nM) and AGN194204 (100 nM) for 16 h. The cells were subsequently infected by VSV (MOI=0.01) and the supernatant was collected at 14 h.p.i. The viral titre was quantified by plaque assay. ( c ) WT and Rxra −/− F9 cells were pretreated with DMSO or AGN194204 (100 nM) for 16 h and subsequently infected with VSV (MOI=0.01). The viral titre of supernatants was quantified by plaque assay at 12 h.p.i. ( d ) Rxra −/− F9 cells stably transfected with pBABE-empty vector (Ctrl) or pBABE-hRXRα (hRXRα) were treated with DMSO or AGN194204 (100 nM) and infected with VSV (MOI=0.01). The viral titre of supernatants was quantified by plaque assay at 12 h.p.i. ( e ) RAW264.7 cells were pretreated with DMSO or 9cRA (100 nM) for 16 h and infected by VSV (MOI=0.01), relative genomic VSV RNA was quantified at 2 and 4 h.p.i. ( f ) RAW264.7 cells were pretreated with DMSO, RXR agonist LG268 (100 nM), AGN194204 (100 nM), VDR agonist Vitamin D (100 nM), LXR agonist GW3965 (100 nM), PPARα agonist GW7647 (100 nM), PPARδ agonist GW1516 (100 nM) or RAR agonist AM580 (100 nM) for 16 h and subsequently infected by VSV (MOI=0.01). The supernatants were collected at 14 h.p.i and viral titre was detected by plaque assay. Data are shown as mean±s.d. ( n =3) of one representative experiment, similar results were obtained in three independent experiments. * P <0.05 and ** P <0.01 (Student’s t -test). Full size image Besides comparing the VSV titre in the supernatant from DMSO- and 9cRA-treated RAW264.7 cells, we also compared VSV genomic RNA and VSV-G protein level. More VSV genomic RNA was detected in 9cRA-treated cells when compared with DMSO-treated cells ( Fig. 2e ). Consistently, more VSV-G protein was observed in both control cells and hRXRα-overexpressing cells after 9cRA treatment ( Supplementary Fig. 2d ). To determine whether RXR agonist and antagonist affect VSV in the first round infection or subsequent infection processes, we used a VSV pseudovirus that has the receptor-binding G protein (VSV-G) replaced by the luciferase reporter (VSVΔG-Luc) enveloped inside VSV-G, called VSVΔG-Luc/G [36] . This pseudovirus can undergo VSV-G-mediated entry but cannot produce its own VSV-G envelope, and hence is only capable of a single-round infection. Significant higher luciferase activity was detected in the cells treated with 9cRA and decreased luciferase activity in the cells treated with HX531 ( Supplementary Fig. 2e ). These results indicate that the RXR agonist and antagonist affect VSV single-round infection. Given that RXRα forms a homodimer or heterodimer to regulate its target genes [6] , [11] , we screened agonists for different RXR potential partners including VDR, LXR, PPARα, PPARδ and RAR. We found that only RAR ligands could promote VSV infection as RXR-specific ligands, which implies that RXR homodimer or RXR/RAR heterodimer mediates the increased host susceptibility to VSV infection ( Fig. 2f ). Taken together, the overexpression of RXRα or ligand activation of RXR increases host susceptibility to VSV infection, while the knockout of RXRα or antagonist inhibition of RXR decreases host susceptibility to VSV infection. Ligand activation of RXRα promotes DNA virus infection Host RXRα expression is downregulated after infection by both RNA and DNA virus. To test if RXRα modulates host response against DNA virus infection as VSV infection, hRXRα-expressing RAW264.7 cells were treated with AGN194204, and infected by DNA viruses, MHV68 and HSV-1. Since MHV68 expressed luciferase, we compared MHV68 infection in DMSO-treated control cells and AGN194204-treated cells by luciferase activity. AGN194204 treatment dramatically increased MHV68 luciferase activity, which indicated the ligand activation of RXR-promoted MHV68 infection ( Fig. 3a ). AGN194204 treatment also increased HSV-1 viral infection significantly as measured by plaque assay ( Fig. 3b ). The overexpression of hRXRα alone slightly increased MHV68 luciferase expression and HSV-1 viral load, whereas treatment with 9cRA significantly increased host cell susceptibility to these viruses ( Fig. 3c,d ). Consistently, the inhibition of RXR activity by HX531 suppressed MHV68 and HSV-1 infections ( Fig. 3c,d ). These results indicate that ligand activation of RXR also increases host susceptibility to DNA viruses. 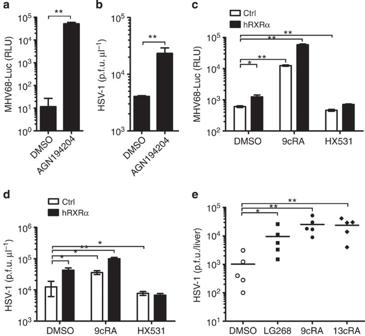Figure 3: Host susceptibility to DNA viral infection after pretreating with RXR agonists and antagonist. (a) hRXRα-overexpressing RAW264.7 cells were treated with DMSO or AGN19420 (100 nM) for 16 h and subsequently infected by luciferase-expressing MHV68 (MHV68-luc; MOI=0.5). Cells were lysed in passive lysis buffer at 24 h.p.i and the luciferase activity was quantified by luminescence assay. (b) hRXRα-overexpressing RAW264.7 cells pretreated with DMSO or AGN19424 (100 nM) and then these cells were infected by HSV-1 (MOI=0.25). Supernatants were collected at 24 h.p.i and the viral titre was quantified by plaque assay. (c) RAW264.7 cells stably expressing pBABE control vector (Ctrl) or pBABE-hRXRα vector (hRXRα) were pretreated with DMSO, 9cRA (100 nM) or HX531 (1 μM) for 16 h, and then infected by MHV68-luc (MOI=0.5). Cells were lysed in passive lysis buffer at 24 h.p.i and the luciferase activity was quantified by luminescence assay. (d) RAW264.7 cells stably expressing Ctrl or hRXRα vector were pretreated with DMSO, 9cRA (100 nM) or HX531 (1 μM) for 16 h, and then infected by HSV-1 (MOI=0.25). Supernatants were collected at 24 h.p.i and the viral titre was quantified by plaque assay. (e) Mice were i.p. injected with DMSO, LG268, 9cRA or 13cisRA (25 μg per mice) daily for 4 days and infected with 107p.f.u. of HSV-1 on day 5. Mice were killed at 5 d.p.i and the livers were harvested, homogenized in media and quantified for viral titres by plaque assay. Data are representative of two independent experiments, *P<0.05 and **P<0.01 (Mann–Whitney test). Data ofa–dare shown as mean±s.d. (n=3) of one representative experiment, similar results were obtained in three independent experiments. *P<0.05 and **P<0.01 (Student’st-test). Figure 3: Host susceptibility to DNA viral infection after pretreating with RXR agonists and antagonist. ( a ) hRXRα-overexpressing RAW264.7 cells were treated with DMSO or AGN19420 (100 nM) for 16 h and subsequently infected by luciferase-expressing MHV68 (MHV68-luc; MOI=0.5). Cells were lysed in passive lysis buffer at 24 h.p.i and the luciferase activity was quantified by luminescence assay. ( b ) hRXRα-overexpressing RAW264.7 cells pretreated with DMSO or AGN19424 (100 nM) and then these cells were infected by HSV-1 (MOI=0.25). Supernatants were collected at 24 h.p.i and the viral titre was quantified by plaque assay. ( c ) RAW264.7 cells stably expressing pBABE control vector (Ctrl) or pBABE-hRXRα vector (hRXRα) were pretreated with DMSO, 9cRA (100 nM) or HX531 (1 μM) for 16 h, and then infected by MHV68-luc (MOI=0.5). Cells were lysed in passive lysis buffer at 24 h.p.i and the luciferase activity was quantified by luminescence assay. ( d ) RAW264.7 cells stably expressing Ctrl or hRXRα vector were pretreated with DMSO, 9cRA (100 nM) or HX531 (1 μM) for 16 h, and then infected by HSV-1 (MOI=0.25). Supernatants were collected at 24 h.p.i and the viral titre was quantified by plaque assay. ( e ) Mice were i.p. injected with DMSO, LG268, 9cRA or 13cisRA (25 μg per mice) daily for 4 days and infected with 10 7 p.f.u. of HSV-1 on day 5. Mice were killed at 5 d.p.i and the livers were harvested, homogenized in media and quantified for viral titres by plaque assay. Data are representative of two independent experiments, * P <0.05 and ** P <0.01 (Mann–Whitney test). Data of a – d are shown as mean±s.d. ( n =3) of one representative experiment, similar results were obtained in three independent experiments. * P <0.05 and ** P <0.01 (Student’s t -test). Full size image Retinoids have been commonly used as drug treatments for skin diseases and various cancers [3] , [11] . 13-cis-retinoic acid (13cRA), also called Isoretinoin, is a ligand for RAR–RXR heterodimer and widely used in clinical settings [37] , [38] , [39] . Like 9cRA, 13cRA also promoted VSV infection in RAW264.7 cells ( Supplementary Fig. 3 ). To test whether retinoids can affect HSV-1 infection in vivo , DMSO or different retinoids were administered by intraperitoneal (i.p.) injection to age and sex-matched mice daily for 4 days. The mice were infected with HSV-1 and the livers were harvested on 5 days post infection. Treatment of RXR ligands, LG268, 9cRA and 13cRA, significantly increased HSV-1 titre in mice livers ( Fig. 3e ). These data are not only supported our in vitro results, but also consistent with the previously reported cases showing that 13cRA may be associated to herpes viral infection [40] , [41] . Together, ligand activation of RXR attenuates host antiviral response against both RNA virus and DNA virus. Activation of RXRα suppressed multiple antiviral genes Since RXRα activation increased host susceptibility to both RNA and DNA viruses, we hypothesized that RXRα caused cellular attenuation of host antiviral response rather than direct enhancement of viral fitness. To test this hypothesis, we performed a microarray to compare the gene expression profiles between DMSO- and 9cRA-treated macrophages after polyI:C transfection. PolyI:C transfection induced 14.88% genes and suppressed 9.42% genes over twofold. These polyI:C-inducible and polyI:C-suppressed genes were considered as polyI:C-responsive genes ( Fig. 4a ). The polyI:C-responseive genes were further grouped into 9cRA-inducible polyI:C-responsive genes ( Fig. 4a and Supplementary Dataset 1 ) and 9cRA-suppressed polyI:C-responsive genes ( Fig. 4a and Supplementary Dataset 2 ). Interestingly, among the 9cRA-suppressed polyI:C-responsive genes, there were multiple type I IFN genes ( Ifnb1 , Ifna2 , Ifna4 , Ifna5 and Ifna9 ) as well as Isg15 ( Fig. 4b ). Given that numerous antiviral genes such as type I IFN and its downstream ISGs can be induced during viral infection and play critical roles in host immune responses against viral infection [25] , [28] , RXR-mediated suppression on these antiviral genes may be responsible for the increased host susceptibility to viral infection. 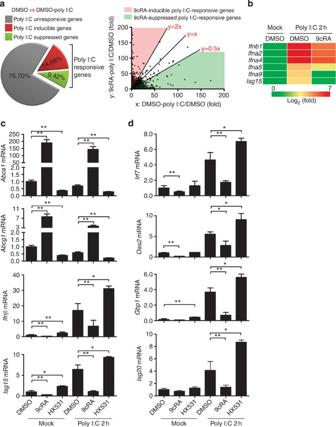Figure 4: Ligand activation of RXR inhibits type I IFN and ISGs. (a,b) RAW264.7 cells were pretreated with DMSO or 9cRA (100 nM) for 16 h and subsequently transfected with 1 μg ml−1polyI:C for 2 h. RNA was extracted and gene expression profile was detected by Affimetrix430.2 Chip. (a) PolyI:C-responsive genes which included polyI:C-inducible genes (DMSO-polyI:C/DMSO>2.0) and polyI:C-suppressed genes (DMSO-polyI:C/DMSO<0.5) were further analysed, the polyI:C-responsive genes can be divided into two groups, 9cRA-inducible polyI:C-responsive genes ((9cRA-polyI:C/DMSO)/(DMSO-polyI:C/DMSO)>2.0) and 9cRA-suppressed polyI:C-responsive genes ((9cRA-polyI:C/DMSO)/(DMSO-polyI:C/DMSO)<0.5). (b) Multiple type I IFN genes were 9cRA-suppressed polyI:C-responsive genes. (c) RAW264.7 cells were pretreated with DMSO, 9cRA (100 nM), or HX531(1 μM) for 16 h and subsequently transfected with 1 μg ml−1polyI:C. RNA was collected 2 h after transfection, the mRNA expression of RXR target genesAbca1,Abcg1and primary antiviral genesIfnβ,Isg15were measured by qPCR. (d) RAW264.7 cells were pretreated as described inc, mRNA expression of ISGs with known antiviral activity,Irf7,Oas2,Gbp1andIsg20were quantified by qPCR. Data ofc,dare shown as mean±s.d. (n=3) of one representative experiment, similar results were obtained in three independent experiments. *P<0.05 and **P<0.01 (Student’st-test). Figure 4: Ligand activation of RXR inhibits type I IFN and ISGs. ( a , b ) RAW264.7 cells were pretreated with DMSO or 9cRA (100 nM) for 16 h and subsequently transfected with 1 μg ml −1 polyI:C for 2 h. RNA was extracted and gene expression profile was detected by Affimetrix430.2 Chip. ( a ) PolyI:C-responsive genes which included polyI:C-inducible genes (DMSO-polyI:C/DMSO>2.0) and polyI:C-suppressed genes (DMSO-polyI:C/DMSO<0.5) were further analysed, the polyI:C-responsive genes can be divided into two groups, 9cRA-inducible polyI:C-responsive genes ((9cRA-polyI:C/DMSO)/(DMSO-polyI:C/DMSO)>2.0) and 9cRA-suppressed polyI:C-responsive genes ((9cRA-polyI:C/DMSO)/(DMSO-polyI:C/DMSO)<0.5). ( b ) Multiple type I IFN genes were 9cRA-suppressed polyI:C-responsive genes. ( c ) RAW264.7 cells were pretreated with DMSO, 9cRA (100 nM), or HX531(1 μM) for 16 h and subsequently transfected with 1 μg ml −1 polyI:C. RNA was collected 2 h after transfection, the mRNA expression of RXR target genes Abca1 , Abcg1 and primary antiviral genes Ifnβ , Isg15 were measured by qPCR. ( d ) RAW264.7 cells were pretreated as described in c , mRNA expression of ISGs with known antiviral activity, Irf7 , Oas2 , Gbp1 and Isg20 were quantified by qPCR. Data of c , d are shown as mean±s.d. ( n =3) of one representative experiment, similar results were obtained in three independent experiments. * P <0.05 and ** P <0.01 (Student’s t -test). Full size image To verify the microarray data and support the hypothesis that ligand activation of RXR suppresses host antiviral gene expression, we performed gene expression assays by qPCR. RAW264.7 cells were pretreated with 9cRA or HX531 overnight and then transfected with polyI:C. Ligand activation of RXR by 9cRA dramatically induced RXR targets genes, Abca1 and Abcg1 . However, the activation of RXR significantly suppressed primary antiviral genes, Ifnβ and Isg15 within 2 h after polyI:C transfection ( Fig. 4c ). Expression of ISGs with antiviral activity, such as Gbp1 , Oas2 , Irf7 and Isg20 , was also suppressed in 9cRA-treated cells ( Fig. 4d ). RXR antagonist, HX531, significantly suppressed Abca1 and Abcg1 expression while upregulated the expression of the antiviral genes tested ( Fig. 4c,d ). Interestingly, 9cRA and HX531 treatment also modulated the basal expression of some of these genes, suggesting that the activation of RXR by endogenous ligands during normal physiological states may suppress antiviral gene activation ( Fig. 4c,d ). Upregulation of type I IFN in Rxra−/− BMMs In addition to RAW264.7 cell lines, we observed similar results in immortalized J2 BMMs. 9cRA treatment suppressed Ifnβ and Ifnα4 expression, while HX531 increased Ifnβ expression in polyI:C-transfected J2 BMMs ( Fig. 5a,b ). Furthermore, we tested type I IFN expression in WT and Rxra−/− primary BMMs. No RXRα could be detected in the lys-Cre-expressed Rxra−/− BMMs ( Fig. 5c ). 9cRA inhibited basal IFNβ and IFNα4 expression, while higher basal IFNβ and IFNα4 were detected in Rxra−/− BMMs ( Fig. 5d,e ). PolyI:C transfection induced IFNβ and IFNα4 in both WT and Rxra−/− BMMs. However, 9cRA significantly suppressed the induction of IFNβ and IFNα4 in WT BMMs, but not in Rxra−/− BMMs ( Fig. 5d,e ). Induction of IFNβ and IFNα4 was also higher in Rxra−/− BMMs than in WT BMMs ( Fig. 5d,e ). Consistently, 9cRA treatment dramatically suppressed IFNβ protein level in WT BMMs whereas Rxra−/− BMMs secreted more IFN than in WT BMMs ( Fig. 5f ). Interestingly, 9cRA also significantly suppressed IFNβ production in Rxra−/− BMMs ( Fig. 5f ), suggesting that ligand activation of RXRβ and RXRγ might also downregulate IFNβ production in primary BMMs. 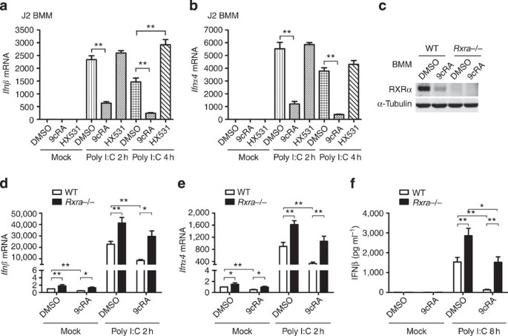Figure 5: RXRα negatively regulates type I IFN expression in immortalized and primary BMMs. (a,b) J2 BMMs were pretreated with DMSO, 9cRA (100 nM) or HX531 (1 μM) for 16 h and subsequently transfected with 1 μg ml−1polyI:C for indicated time. The mRNA expression ofIfnβ(a) andIfnα4(b) were measured by qPCR. (c) Immunoblot of RXRα in the WT andRxra−/− BMMs that pretreated with DMSO or 9cRA (100 nM) for 24 h. (d–f) WT andRxra−/− BMMs pretreated with DMSO or 9cRA (100 nM) for 24 h, then the cells were transfected with 1 μg ml−1polyI:C for 2 h.Ifnβ(d) andIfnα4(e) mRNA expression were measured by qPCR. IFNβ protein level were detected by enzyme-linked immunosorbent assay after 8 h polyI:C transfection. Data ofa,bandd–fare shown as mean±s.d. (n=3) of one representative experiment, similar results were obtained in three independent experiments. *P<0.05 and **P<0.01 (Student’st-test). Data ofcare representative of three independent experiments. See alsoSupplementary Fig. 7of uncropped blot ofc. Figure 5: RXRα negatively regulates type I IFN expression in immortalized and primary BMMs. ( a , b ) J2 BMMs were pretreated with DMSO, 9cRA (100 nM) or HX531 (1 μM) for 16 h and subsequently transfected with 1 μg ml −1 polyI:C for indicated time. The mRNA expression of Ifnβ ( a ) and Ifnα4 ( b ) were measured by qPCR. ( c ) Immunoblot of RXRα in the WT and Rxra −/− BMMs that pretreated with DMSO or 9cRA (100 nM) for 24 h. ( d – f ) WT and Rxra −/− BMMs pretreated with DMSO or 9cRA (100 nM) for 24 h, then the cells were transfected with 1 μg ml −1 polyI:C for 2 h. Ifnβ ( d ) and Ifnα4 ( e ) mRNA expression were measured by qPCR. IFNβ protein level were detected by enzyme-linked immunosorbent assay after 8 h polyI:C transfection. Data of a , b and d – f are shown as mean±s.d. ( n =3) of one representative experiment, similar results were obtained in three independent experiments. * P <0.05 and ** P <0.01 (Student’s t -test). Data of c are representative of three independent experiments. See also Supplementary Fig. 7 of uncropped blot of c . Full size image Taken together, these genetic and pharmacological studies provide evidence that RXR activation negatively regulates antiviral genes including type I IFN in macrophages. RXRα inhibits type I IFN independent of IFNAR signalling Generally, viral infections directly trigger expression of primary antiviral genes such as IFNβ and ISG15, and induction of IFNβ amplifies expression of antiviral effectors through autocrine or paracrine action [27] . To investigate the mechanism for the suppression of type I IFN by ligand activation of RXR, we used IFNαβ receptor deficient BMMs ( Ifnar1−/− ) to test if ligand activation of RXR regulated primary type I IFN production or IFNAR downstream signalling-dependent type I IFN production positive feedback. Therefore, we pretreated Ifnar1−/− BMMs with 9cRA and HX531 and activated them by polyI:C transfection, expression of Ifnβ , Isg15 , and some ISGs were measured by qPCR. Ligand activation of RXR by 9cRA and LG268 significantly downregulated polyI:C-induced Ifnβ and Isg15 in Ifnar1−/− BMMs ( Fig. 6a,b and Supplementary Fig. 4a,b ). No induction of Oas2 , Gbp1 , Irf7 and Isg20 was observed in polyI:C-activated Ifnar1−/− BMMs ( Supplementary Fig. 4c ), which support that induction of these ISGs is type I IFN-dependent. These results suggest that ligand activation of RXR modulates the expression of a specific set of primary antiviral genes including IFNβ independent of IFNAR signalling, though we cannot exclude that RXR regulates IFNAR downstream signalling simultaneously. 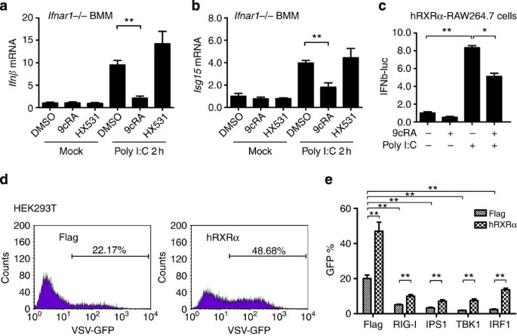Figure 6: RXRα inhibits type I IFN transcription independent of IFNAR signalling. (a,b)Ifnar−/−BMMs were pretreated with DMSO, 9cRA (100 nM) or HX531 (1 μM) for 24 h and transfected with 1 μg ml−1polyI:C.IfnβandIsg15mRNA were quantified by qPCR. Data are shown as mean±s.d. (n=3) of one representative experiment, similar results were obtained in three independent experiments, **P<0.01 (Student’st-test). (c) hRXRα-stably transfected RAW264.7 cells were transfected with IFNβ promoter luciferase reporter (IFNβ-luc) and treated with DMSO or 9cRA (100 nM) for 9 h before stimulation with polyI:C (5 μg ml−1). The lysates were collected 20 h after polyI:C stimulation and luciferase reporter activity was measured by luminescence assay. RLU is represented as mean±s.d. (n=6) and is representative of three experiments. *P<0.05 and **P<0.01 (Student’st-test). (d) Flag or hRXRα vector was transfected into HEK293T cells for 24 h, subsequently the transfected cells were infected by VSV-GFP (MOI=0.01) for 8 h, fluorescence-activated cell sorting (FACS) assay was performed to detect the GFP-positive cells as VSV-infected cells. Data are representative of three independent experiments. (e) Flag or hRXRα was co-transfected with RIG-I and TLR3 pathway components for 24 h into 293T cells, subsequently the transfected cells were infected by VSV-GFP (MOI=0.01) for 8 h, FACS assay was performed to detect the VSV virus in the cells. The ratio of GFP-positive cell is represented as mean±s.d. (n=3) and is representative of three experiments,P<0.01 (Student’st-test). Figure 6: RXRα inhibits type I IFN transcription independent of IFNAR signalling. ( a , b ) Ifnar−/− BMMs were pretreated with DMSO, 9cRA (100 nM) or HX531 (1 μM) for 24 h and transfected with 1 μg ml −1 polyI:C. Ifnβ and Isg15 mRNA were quantified by qPCR. Data are shown as mean±s.d. ( n =3) of one representative experiment, similar results were obtained in three independent experiments, ** P <0.01 (Student’s t -test). ( c ) hRXRα-stably transfected RAW264.7 cells were transfected with IFNβ promoter luciferase reporter (IFNβ-luc) and treated with DMSO or 9cRA (100 nM) for 9 h before stimulation with polyI:C (5 μg ml −1 ). The lysates were collected 20 h after polyI:C stimulation and luciferase reporter activity was measured by luminescence assay. RLU is represented as mean±s.d. ( n =6) and is representative of three experiments. * P <0.05 and ** P <0.01 (Student’s t -test). ( d ) Flag or hRXRα vector was transfected into HEK293T cells for 24 h, subsequently the transfected cells were infected by VSV-GFP (MOI=0.01) for 8 h, fluorescence-activated cell sorting (FACS) assay was performed to detect the GFP-positive cells as VSV-infected cells. Data are representative of three independent experiments. ( e ) Flag or hRXRα was co-transfected with RIG-I and TLR3 pathway components for 24 h into 293T cells, subsequently the transfected cells were infected by VSV-GFP (MOI=0.01) for 8 h, FACS assay was performed to detect the VSV virus in the cells. The ratio of GFP-positive cell is represented as mean±s.d. ( n =3) and is representative of three experiments, P <0.01 (Student’s t -test). Full size image We took the advantage of the IFNβ promoter luciferase reporter (IFNβ-luc) to test if 9cRA suppressed IFNβ transcriptionally or post-transcriptionally. We found that 9cRA treatment significantly suppressed the IFNβ-luc activity triggered by transfection of polyI:C ( Fig. 6c ), which suggests that ligand activation of RXR inhibits IFNβ transcription. VSV triggered host cell to produce type I IFN mainly through RIG-I and TRIF pathways, overexpression of the components of RIG-I and TRIF pathways can facilitate the host cells to clear the infected VSV. In HEK293T cells, more VSV-infected cells can be observed after overexpression of hRXRa, similar to the results with RAW264.7 ( Fig. 6d ). Overexpression of RIG-I, IPS1, TBK1 or IRF1 facilitated host cells to clear VSV; however, co-expression of hRXRα with these genes attenuated VSV clearance by host cells ( Fig. 6e ). Considering that transfection of RIG-I, IPS1, TBK1 or IRF1 triggered type I IFN in HEK293T cells, these data not only support the role of RXRα in the increase of host susceptibility to VSV infection by type I IFN suppression, but also suggest RXRα potentially regulates type I IFN production downstream of TBK1. Activation of RXR inhibit β-catenin nuclear translocation Transfected polyI:C or infected VSV could be recognized by RIG-I and TLR3. RIG-I and TLR3 recruit the adaptor molecule IPS1 and TRIF, respectively. Both IPS1 and TRIF facilitate TBK1 and IRF3 phosphorylation, which leads to IRF3 dimerization and translocation into nucleus to drive IFNβ transcription [24] , [25] , [26] . RIG-I and TRIF pathway components triggered IFNβ promoter activity in HEK293T cells. However, the co-transfection of hRXRα significantly suppressed the IFNβ promoter activity activated by TRIF, RIG-I, IPS1, TBK1 and IRF3 ( Fig. 7a ). Considering that if hRXRα only regulates the expression or activity of RIG-I, IPS1 or TBK1, IFNβ promoter activity activated by the overexpression of IRF3 should not be affected. Therefore, these data suggest that RXR inhibits IFNβ downstream of IRF3, for example, IFNβ enhanceosome, although we cannot exclude the possibility that RXR concurrently regulates IFNβ production upstream of IRF3. 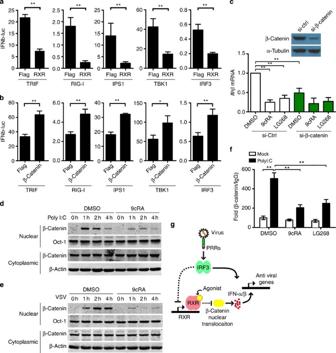Figure 7: Ligand activation of RXRα inhibits β-catenin nuclear translocation. (a,b) IFNβ-luc reporter were co-transfected with flag or hRXRα, and indicated components of RIG-I and TLR3 signalling pathway into 293T cells for 24 h, the luciferase activity of the lysate was detected (a). IFNβ-luc reporter were co-transfected with flag or β-catenin, and indicated components of RIG-I and TLR3 signalling pathway into 293T cells for 24 h, the luciferase activity of the lysate was detected (b). IFNβ-luc activity is represented as mean±s.d. (n=6) and is representative of three experiments.*P<0.01 (Student’st-test). (c) RAW264.7 cells were transfected with 20 nM control siRNA (si-Ctrl) or siRNA targeting β-catenin (si-β-catenin). Twenty-four hours post transfection, the cells were treated with DMSO, 9cRA (100 nM) or LG268 (100 nM) for another 16 h, and then these cells were transfected with 1 μg ml−1polyI:C for 2 h,IfnβmRNA expression were measured by qPCR. β-catenin protein level was quantified by immunoblot after the cells being transfected with siRNA for 24 h, α-tubulin was shown as a loading control. (d,e) J2 BMMs were pretreated with DMSO or 9cRA (100 nM) for 16 h, and then the cells were transfected with 3 μg ml−1polyI:C (d) or infected by 1 MOI VSV (e) for indicated time. Nuclear and cytoplasmic β-catenin were detected by immunoblot, Oct1 and β-actin were shown as loading controls. Data are representative of three independent experiments. (f) J2 BMMs were pretreated with DMSO, 9cRA (100 nM) or LG268 (100 nM) for 16 h, and then the cells were transfected with 3 μg ml−1polyI:C for 2 h, the binding ofIfnb1promoter region with β-catenin (or IgG) was detected by ChIP-qPCR. The data was shown as fold change of β-catenin/IgG. Data ofcandfare shown as mean±s.d. (n=3) of one representative experiment, similar results were obtained in three independent experiments, **P<0.01 (Student’st-test). Data ofd,eare representative of three independent experiments. See alsoSupplementary Fig. 7of uncropped blot ofd,e. (g) Working model for RXRα regulating host antiviral responses. Dash line: indirect regulation. Figure 7: Ligand activation of RXRα inhibits β-catenin nuclear translocation. ( a , b ) IFNβ-luc reporter were co-transfected with flag or hRXRα, and indicated components of RIG-I and TLR3 signalling pathway into 293T cells for 24 h, the luciferase activity of the lysate was detected ( a ). IFNβ-luc reporter were co-transfected with flag or β-catenin, and indicated components of RIG-I and TLR3 signalling pathway into 293T cells for 24 h, the luciferase activity of the lysate was detected ( b ). IFNβ-luc activity is represented as mean±s.d. ( n =6) and is representative of three experiments. * P <0.01 (Student’s t -test). ( c ) RAW264.7 cells were transfected with 20 nM control siRNA (si-Ctrl) or siRNA targeting β-catenin (si-β-catenin). Twenty-four hours post transfection, the cells were treated with DMSO, 9cRA (100 nM) or LG268 (100 nM) for another 16 h, and then these cells were transfected with 1 μg ml −1 polyI:C for 2 h, Ifnβ mRNA expression were measured by qPCR. β-catenin protein level was quantified by immunoblot after the cells being transfected with siRNA for 24 h, α-tubulin was shown as a loading control. ( d , e ) J2 BMMs were pretreated with DMSO or 9cRA (100 nM) for 16 h, and then the cells were transfected with 3 μg ml −1 polyI:C ( d ) or infected by 1 MOI VSV ( e ) for indicated time. Nuclear and cytoplasmic β-catenin were detected by immunoblot, Oct1 and β-actin were shown as loading controls. Data are representative of three independent experiments. ( f ) J2 BMMs were pretreated with DMSO, 9cRA (100 nM) or LG268 (100 nM) for 16 h, and then the cells were transfected with 3 μg ml −1 polyI:C for 2 h, the binding of Ifnb1 promoter region with β-catenin (or IgG) was detected by ChIP-qPCR. The data was shown as fold change of β-catenin/IgG. Data of c and f are shown as mean±s.d. ( n =3) of one representative experiment, similar results were obtained in three independent experiments, ** P <0.01 (Student’s t -test). Data of d , e are representative of three independent experiments. See also Supplementary Fig. 7 of uncropped blot of d , e . ( g ) Working model for RXRα regulating host antiviral responses. Dash line: indirect regulation. Full size image β-catenin, as a co-activator in the pathway for IRF3-mediated production of type I IFN, regulates the host antiviral response against Listeria monocytogenes , VSV, Sendai virus and HSV-1 (refs 28 , 29 , 30 , 31 ). Consistent with these studies, co-transfection with β-catenin significantly upregulated the IFNβ promoter activity activated by TRIF, RIG-I, IPS1, TBK1 and IRF3 ( Fig. 7b ). We hypothesized that hRXRα inhibits IFNβ enhanceosome by regulating β-catenin activity. By transfecting an efficient short interfering RNA (siRNA) to interfere with endogenous β-catenin in J2 BMMs, we found that polyI:C-triggered IFNβ expression was attenuated after the knockdown of β-catenin, and the inhibition of IFNβ induction by 9cRA and LG268 was almost abolished by the siRNA targeting β-catenin ( Fig. 7c ). Since activated β-catenin enters into the nucleus and forms a complex to drive IFNβ expression [28] , [29] , we compared the nuclear β-catenin between DMSO- and RXR agonists-treated macrophages. Both polyI:C transfection and VSV infection did not change cytoplasmic β-catenin levels but increased nuclear β-catenin significantly. 9cRA and LG268 treatment suppressed β-catenin nuclear translocation compared with DMSO-treated controls ( Fig. 7d,e and Supplementary Fig. 5 ). These results showed that RXR inhibited β-catenin translocation and led to the downregulation of type I IFN expression. In addition, by using the β-catenin reporter system [42] , we found that 9cRA and LG268 treatment inhibited the transcriptional activity of β-catenin in RAW264.7 cells, which was consistent with that ligand activation of RXR blocked β-catenin nuclear translocation ( Supplementary Figs 6 and 7 ). Transfection of polyI:C significantly increased the binding of β-Catenin to Ifnb1 promoter region ( Fig. 7f ); however, ligand activation of RXR by 9cRA or LG268 attenuated the binding between β-catenin and Ifnb1 promoter triggered by polyI:C transfection ( Fig. 7f ). In summary, our data along with our published data showing that IRF3 downregulates RXR expression, illustrating that IRF3 not only activates antiviral gene expression directly, but also indirectly through the alleviation the RXR-β-catenin-dependent suppressive pathway to achieve optimal antiviral immune response ( Fig. 7g ). RXRα is a key player in the cellular and whole-body metabolic and immune processes, and our previous study has suggested that the downregulation of RXRα expression during viral infections would alter drug metabolisms leading to metabolic diseases such as Reye’s Syndrome [18] . In our current study, we demonstrated that the downregulation of RXRα is an innate immune defence mechanism important for host against viral infections. As RXR agonists and antagonists are increasingly used in clinics, our studies raises an open question about the potential differential effects of these drugs on patients with or without viral infections. Previous studies have indicated that RXR heterodimers control host against Listeria monocytogenes and Mycobaterium tuberculosis infection [22] , [23] . A recent study suggested that RXRα is an important factor in the gene network involved in host defence against Leishmania donovani [43] . In addition to controlling host immune responses to bacterial and parasitic infections, we have shown here that RXRα overexpression or ligand activation increases host cell susceptibility to VSV, MHV68 and HSV-1 infection. RXRα-deficient or RXRα antagonist-treated cells were more resistant to these viral infections. Moreover, RXR agonist-treated mice were more susceptible to HSV-1 infection. These results suggest that RXR signalling negatively regulates host antiviral response, and the downregulation of RXRα benefits the host cellular immunity against viral infections. This study has described a unique crosstalk between host antiviral response and nuclear receptor RXR, suggesting that NRs may differentially affect host innate immunity against different pathogens. Type I IFN and its downstream ISGs are critical for host defence against viruses [27] . Our microarray analysis and qPCR data indicated that multiple type I IFN genes and ISGs were suppressed in RXR agonist-treated macrophages. There was also increased basal and polyI:C-induced IFNβ expression in Rxra−/− BMMs than WT BMMs, providing the evidence that RXR signalling negatively regulates host antiviral response by inhibiting type I IFN and ISGs expression. Since ligand activation of RXR inhibits IFNβ promoter activity independent of IFNαβ receptor and RXRα might suppress IFNβ transcription downstream of the IRF3 transcription factor, we hypothesized that RXRα regulates the components of IFNβ enhanceosome. β-catenin has been reported as a co-activator of IFNβ enhanceosome during viral and bacterial infection [29] , [30] , [31] . IFNβ reporter assays also suggest that β-catenin is a potential target to be regulated by RXR signalling. Ligand activation of RXR inhibits the transcription activity of β-catenin in macrophages, which is consistent with the previous study performed in HEK293 cells [44] . Knockdown of β-catenin almost abolished the RXR-dependent suppressive effect on IFNβ induction by polyI:C. By detecting the cytoplasmic and nuclear β-catenin, we observed that ligand activation of RXR suppressed nuclear β-catenin, while it had no effect on cytoplasmic β-catenin. Ligand activation of RXR also attenuated the binding of β-Catenin to Ifnb1 promoter. These data suggested that RXR could suppress β-Catenin nuclear translocation and subsequent type I IFN induction. However, the detail for the regulation of β-catenin by RXR needs to be further investigated, which is likely through an indirect mechanism as our preliminary results showed that the suppression of β-catenin nuclear translocation required overnight RXR agonist treatment and was also sensitive to new protein synthesis inhibitor, cycloheximide. Our study supports a model by which modulation of RXR controls host antiviral immunity. During the absence of infection, RXR is constitutively expressed and can be activated by multiple endogenous RXR ligands, such as 9cRA, docosahexaenoic acid, oleic acid and phytanic acid, to suppress basal and inducible IFN expression. However, during viral infection, the host cell downregulates RXRα expression in an IRF3-dependent manner to achieve optimal IFN expression. The major function of IRF3 is known to directly bind to the promoter region of primary type I IFN genes such as IFNβ to initiate IFN response. Our study, therefore, reveals an indirect function of IRF3 in IFN induction through relieving RXR-mediated suppression of IFN genes. After infection, to avoid excess type I IFN production, RXR expression level is restored by host cells and exerts its suppressive function on the type I IFN induction in the presence of the RXR endogenous ligands. Therefore, RXR not only maintains the basal type I IFN and modulates the host antiviral response, but also regulates the resolution of infection. Retinoids and rexinoids are frequently used in the clinical setting as treatment for cancer, inflammatory skin diseases and acne [7] , [11] , [15] . Accutane and Isotretinoin have been approved to treat acne and cancer [37] , [38] , [39] . Targretin has been used in therapy for the treatment of cutaneous T-cell lymphoma and is in clinical trials for the treatment of breast and lung cancer [15] . In addition to their applications in cancer, rexinoids are being tested in the treatment of diabetes, obesity, atherosclerosis and other cardiovascular indications and inflammatory diseases [3] , [11] . On the other hand, treatment with rexinoids or retinoids raises plasma triglyceride levels, suppresses the thyroid hormone axis and induces hepatomegaly [11] , [15] . Our results show that retinoids or rexinoids treatment increases susceptibility to HSV-1 infection in mice and support clinical reports of association of Isotretinoin with herpetic infections [40] , [41] . However, further investigation is needed to evaluate the overall impact of the RXR agonists on virally infected patients. Nonetheless, our data present the potential application of RXR antagonist in treatment of viral infection-related diseases. Mice and reagents C57BL/6 male mice (6–8 weeks of age) and Ifnar1−/− mice were from the Jackson Laboratory. All mice experiments were performed in accordance with guidelines from the University of California, Los Angeles, Institutional Animal Care and Use Committee. HEK293T and RAW264.7 cells were purchased from ATCC and cultured in Dulbecco's modified Eagle's medium (DMEM) with 10% fetal bovine serum (FBS) and 1% penicillin/streptomycin. RXRα fl/fl (WT) and LysM-Cre + /RXRα fl/fl ( Rxra−/− ) mice bone marrows were overnight shipped from Dr Mercedes Ricote’s Lab (Spain) [13] . WT, Ifnar1−/− and Rxra−/− BMMs were differentiated as described previously [45] . WT and Rxra−/− F9 embryocarcinoma cells, as well as RXR-specific agonists AGN194204 and LG268 were obtained from Dr Peter Tontonoz’s Lab (University of California, Los Angeles). HX531 was obtained from Dr Hiroyuki Kagechika’s lab (Tokyo Medical and Dental University). 9cRA and 13cRA were purchased from Sigma-Aldrich. All compounds for in vitro treatment were solubilized in DMSO. PolyI:C and polydA:dT were from InvivoGen. Antibody against α-tubulin was from Sigma-Aldrich. Anti-VSV-G (P5D4) and anti-Oct1 (C-21) antibodies were from Santa Cruz Biotechnology. Anti-RXRα (D6G10), anti-β-Actin (13E5) and anti-β-Catenin (D10A8) were from Cell Signaling Technology. Anti-GAPDH (GT239) was from GeneTex. Stable cell lines and BMM immortalization hRXRα-flag, hRXRαK108R-flag and hRXRαΔEF-flag were cloned into pBABE retroviral vector to make WT or mutated hRXRα pBABE constructs. These constructs or pBABE-empty vector was co-transfected with packaging vectors psiA into HEK293T cells for 48 h. The viral supernatants were collected and used to transduce control or hRXRα (WT and its mutants) into RAW264.7 or F9 embryocarcinoma cells. The transduced cells were selected by puromycin (2 μg ml −1 ) for 2 weeks, and then the transformed cells were stable cell lines. For J2 virus-immortalized macrophages (J2 BMMs), a cell line transformed by retrovirus expressing v-raf and c-myc, was established (called GG2EE) and grown in RPMI1640 (10 mM HEPES PH7.8, 10% FBS, 1% Pen/strep) [46] , [47] . The supernatant containing J2 viruses was harvested and filtered through 0.22 μm filter. Bone marrow cells were infected with the J2 virus and immortalized as J2 BMMs. Viral mimics and siRNA transfection For activating cells by transfection with polyI:C and polydA:dT in a six-well plate, 5 μl of Lipofectamine 2000 (Life Technolgies) was diluted in 200 μl Opti-MEM for 5 min. PolyI:C or polydA:dT (2 μg) were diluted in 200 μl Opti-MEM. Mixed the above Lipofectamine 2000 solution and polyI:C (or polydA:dT) solution, and incubated in room temperature for 15 min. Subsequently, the mixed solution was added into the cells with 1.6 ml fresh medium. Jet-PEI (Polyplus Transfection) was used to transfect plasmids into HEK293T cells according to the manufacturer’s instructions. siRNA target mouse β-catenin (SMARTpool: siGENOME Ctnnb1 siRNA) and its control were purchased from Dharmacon. RAW264.7 cells were transfected with 20 nM control or β-catenin by using INTERFERin (Polyplus Transfection) according to the manufacturer’s instructions. Ligand activation and viral Infection RAW264.7 cells were plated in a six-well format at 6 × 10 5 and treated with DMSO, RXR agonists or RXR antagonist for 16–24 h. Replication competent VSV-GFP was graciously provided by Dr Glen Barber and MHV68-luc was from Dr Ren Sun Lab (University of California, Los Angeles). Viruses were propagated as described previously [48] , [49] . Cells were infected with VSV (multiplicity of infection, MOI=0.01) in media for 1 h and replenished with DMEM with 1% FBS. Supernatants were collected between 12 and 16 h.p.i. MHV68-luc infection was quantified by firefly luciferase assay kit (Promega Inc.). VSV-G pseudotyped virus containing renilla luciferase reporter was a gift from Dr Benhur Lee (University of California, Los Angeles). Infections were performed similarly and quantified by renilla luciferase kit (Promega Inc.). Flow cytometry was performed to detect the VSV-GFP in HEK293T cells on FACScaliber (BD Biosciences) with standard compensation and the data was analysed using CellQuest (BD Biosciences). Plaque assay Standard plaque assay was performed on a monolayer of Vero cells. Briefly, Vero cells were seeded at 2.5 × 10 5 cells per well in standard 12-well plates. Tenfold serial dilutions of VSV viral supernatants were made. Vero cells were infected with diluted supernatants for 1 h and resuspended in 1% FBS with 0.6% low-melt point agarose in DMEM overnight. The agarose was removed by suction and stained with 0.05% crystal violet, 40% EtOH, in PBS. HSV-1 (MOI=0.25) and MHV68-luc (MOI=1) infections were done by a similar way. HSV-1 plaque assay took 60 h for plaques to form and were stained the same way. RNA isolation, reverse transcrption and real time qPCR Biological triplicates of RAW264.7 cells were pretreated with 9cRA (100 nM) or HX531 (1 μM) for 16 h and subsequently transfected with polyI:C (1 μg ml −1 ). Cells were lysed in Trizol and RNA was isolated by standard isopropanol precipitation. RNA was quantified by spectrometry. cDNA was generated using 1 μg of RNA with IScript reverse transcription kit (BioRad) according to the manufacturer’s instructions with either random hexamers or VSV N1 (5′ GATAGTACCGGAGGATTGACGACTA-3′) as primers. qPCR analysis was done using the iCycler thermocycler (Bio Rad). qPCR was performed by using Sensimix SYBR & Fluorescein Kit (Bioline) according to the manufacturer’s instructions. Expression values were normalized to L32 control and fold induction was normalized to untreated control by using 2 −ΔΔ C t Method [50] . Gene primer sequences used were: Rxra : 5′-ATGGACACCAAACATTTCCTGC-3′ and 5′-CCAGTGGAGAGCCGATTCC-3′; VSV: 5′-GATAGTACCGGAGGATTGACGACTA-3′ and 5′-CTTACCGAGCCTACCAAACT; Abca1 : 5′-GCTTGTTGGCCTCAGTTAAGG-3′ and 5′-GTAGCTCAGGCGTACAGAGAT-3′; Abcg1 : 5′-GGAGTACGGGGATCAGAACA-3′ and 5′-AAAGAAACGGGTTCACATCG-3′; Ifnb1 : 5′-CAGCTCCAAGAAAGGACGAAC-3′ and 5′-GGCAGTGTAACTCTTCTGCAT-3′; Ifna4 : 5′-TGATGAGCTACTACTGGTCAGC-3′ and 5′-GATCTCTTAGCACAAGGATGGC-3′; Isg15 : 5′-CAGGACGGTCTTACCCTTTCC-3′ and 5′-AGGCTCGCTGCAGTTCTGTAC-3′; Gbp1 : 5′-CAGGGTAGACAATGGGCAGT-3′ and 5′-CACAGTAGGCTGGAGCATGA-3′; Oas2 : 5′-GGTGAGGGTCCCATAACCTT-3′ and 5′-AGTCCACCAGAGCCTGCTTA-3′; Irf7 : 5′-ACAGGGCGTTTTATCTTGCG-3′ and 5′-TCCAAGCTCCCGGCTAAGT-3′; Isg20 : 5′-CCATGGACTGTGAGATGGTG-3′ and 5′-CTCGGGTCGGATGTACTTGT-3′; L32 : 5′-AAGCGAAACTGGCGGAAAC-3′ and 5′-TAACCGATGTTGGGCATCAG-3′. Assay of luciferase reporter gene expression HEK293T or hRXRα-RAW264.7 cells were co-transfected with a mixture of IFNβ firefly luciferase reporter plasmids (IFNβ-luc), pRL-TK renilla luciferase plasmids and other indicated constructs by using Jet-PEI (Polyplus Transfection) according to the manufacturer’s instructions. Luciferase activity was measured with the Dual-Luciferase Reporter Assay System (Promega Inc.) as described [51] , [52] . Data were normalized for transfection efficiency by division of firefly luciferase activity with renilla luciferase activity. Nuclear and cytoplasmic protein separation and western blot Cells were harvested and lysed with M-PER Protein Extraction Reagent (Pierce, Rockford, IL) supplemented with protease inhibitor cocktail (Calbiochem). Nuclear protein was extracted using NE-PER nuclear and Cytoplasmic Extraction Reagents (Pierce). Protein concentrations of the extracts were measured with bicinchoninic acid assay (Pierce) and equalized with the extraction reagent. Equal amounts of the extracts were used for immunoprecipitation, or loaded and subjected to SDS-polyacrylamide gel electrophoresis, transferred onto nitrocellulose membranes and then blotted as described previously [51] , [52] . HSV-1 infection in vivo The RXR agonists LG268, 9cRA and 13cRA were dissolved in DMSO (25 μg μl −1 ). DMSO or RXR (1 μl) agonist solution was diluted in 100 μl saline for each mice injection. WT C57/BL6 were injected i.p. with DMSO, LG268, 9cRA or 13cRA (25 μg per mice) daily for 4 days ( n =5). The mice were infected with HSV-1(10 7 p.f.u. of Strain 17) on day 5. Mice were killed 5 d.p.i and the livers were harvested, homogenized in media and quantified for viral titres by standard plaque assay. Affimetrix microarray Gene expression profiling of RAW264.7 cells pretreated with DMSO or 9cRA and activated by polyI:C transfection was done on an Affymetrix 430.2 Chip by the UCLA Genotyping and Array. ELISA and ChIP assay IFNβ in culture supernatant was quantified with VeriKine Mouse Interferon Beta ELISA Kit (PBL interferon source) according to the manufacturer’s instructions. Chromatin immunoprecipitation (ChIP) assays were performed according to the protocol of the ChIP assay kit (Magna ChIP HiSens kit, catalogue No. 17-10460, Millipore). β-catenin (D10A8) XP Rabbit mAb (#8480) from Cell Signaling Technology was used for ChIP assay at the concentration of 2 μg antibody per reaction. Primer pair specific for the Ifnb1 promoter region has been described [53] . Ifnb1 promoter region in both input and immunoprecipitated genomic DNA was detected by qPCR. The percentage of Ifnb1 promoter region immunoprecipitated by β-catenin or its isotype IgG relative to input DNA was calculated, the data was shown the enrichment of the Ifnb1 promoter region by β-catenin. How to cite this article: Ma, F. et al. Retinoid X receptor α attenuates host antiviral response by suppressing type I interferon. Nat. Commun. 5:5494 doi: 10.1038/ncomms6494 (2014). Accession codes: Microarray data was deposited in GEO (Accession number: GSE62107 ).